Direct and selective access to amino-poly(phenylene vinylenes)s with switchable properties by dimerizing polymerization of aminoaryl carbenes Despite the ubiquity of singlet carbenes in chemistry, their utility as true monomeric building blocks for the synthesis of functional organic polymers has been underexplored. In this work, we exploit the capability of purposely designed mono- and bis-acyclic amino(aryl)carbenes to selectively dimerize as a general strategy to access diaminoalkenes and hitherto unknown amino-containing poly(p-phenylene vinylene)s (N-PPV’s). The unique selectivity of the dimerization of singlet amino(aryl)carbenes, relative to putative C-H insertion pathways, is rationalized by DFT calculations. Of particular interest, unlike classical PPV’s, the presence of amino groups in α-position of C=C double bonds in N-PPV’s allows their physico-chemical properties to be manipulated in different ways by a simple protonation reaction. Hence, depending on the nature of the amino group (iPr 2 N vs . piperidine), either a complete loss of conjugation or a blue-shift of the maximum of absorption is observed, as a result of the protonation at different sites (nitrogen vs . carbon). Overall, this study highlights that singlet bis-amino(aryl)carbenes hold great promise to access functional polymeric materials with switchable properties, through a proper selection of their substitution pattern. Singlet carbenes have witnessed tremendous developments since the isolation of the first stable carbenes by Bertrand et al. [1] in 1988 and Arduengo et al. [2] in 1991. In particular, a great variety of stable singlet carbenes has been prepared over the past 30 years [3] , [4] , [5] , [6] , [7] , [8] . Most examples reported to date feature a cyclic backbone and are thermodynamically stabilized thanks to the presence of one or two amino groups next to the carbene center, as highlighted with cyclic (alkyl)(amino)carbenes [9] and N -heterocyclic carbenes [10] , respectively. Nevertheless, some acyclic mono-aminocarbenes (MACs) have also been isolated [11] , [12] , providing that the carbene center benefits from sufficient steric protection. Indeed, in the absence of sufficient kinetic stabilization, dimerization of the carbene into the corresponding tetra-aminoethylene and diaminoethylene has been observed in the case of (cyclic) di-amino and (acyclic) mono-aminocarbenes, respectively [13] , [14] , [15] , [16] , [17] . Such a dimerization reaction has been proposed to occur following a non-least motion pathway, involving the attack of the occupied in-plane σ orbital of one carbene onto the out-of-plane 2p π orbital of a second carbene [15] , [18] , [19] , [20] . In fact, dimerization, as well as the reverse process reforming the carbene, appear to be most generally catalyzed by electrophilic impurities [21] , [22] , [23] , [24] . While this dimerization reaction is often considered as deleterious for the isolation of carbenes, it eventually offers a powerful way to construct C=C double bonds. Surprisingly, in the context of polymer chemistry, dimerization of bis-carbenes has received little attention so far [25] , [26] , [27] , [28] . Bielawski et al. reported that some bis-benzimidazol-2-ylidenes, generated by deprotonation of the corresponding bis-benzimidazoliums, could undergo such a dimerization/polymerization, forming a class of thermally reversible dynamic covalent conjugated polymers [29] , [30] , [31] , though showing a low conjugation across the aryl spacer [32] in addition to be rather air-sensitive. Formal polymerization by dimerization of non-heteroatom-stabilized bis-(aryl)carbenes, generated by decomposition of corresponding bis-diazo compounds, has also been reported [33] , [34] , [35] , [36] . Depending on the nature of the catalyst, either poly(phenylene vinylene)s (PPV’s) or poly(aryl azine)s could be achieved, upon extrusion or retention of N 2 , respectively. PPV’s represent an attractive class of highly stable, non-dynamic, and fluorescent polymeric semi-conductors that have received considerable attention [37] , [38] . Thus, besides the aforementioned diazo route, a variety of different synthetic approaches to PPV-like materials, involving either a step-growth or a chain-growth polymerization route, have been developed [39] , [40] . In general, related synthetic methods provide safer access to PPV’s, in comparison to those involving the decomposition of diazo-containing precursors. They also allow the structural diversity of PPV’s to be significantly broadened (in contrast, diazo precursors feature electron-withdrawing substituents only) [41] . While specific groups have been incorporated into the aromatic moiety of PPV’s as a means to increase their solubility and facilitate their processability, introduction of heteroatoms directly linked to the double bond would yield PPV’s with original optoelectronic properties [42] , [43] . These properties may even be finely tuned upon post-chemical modification of the basic amino groups [44] in 1,2-position of the double bonds, in contrast to the behavior of PPV’s free of such α-amino substituents. We thus reasoned that these amino-PPV’s, denoted as N-PPV’s, i.e. containing two amino groups directly connected to the double bonds, could be accessible following a direct and selective dimerizing polymerization approach involving hitherto unknown bis-aminoaryl carbenes (see Fig. 1 ). Fig. 1: Synthetic strategy to amino-poly(phenylene vinylene)s (N-PPV’s). NPPV’s via dimerizing polymerization of in situ generated bis-amino(aryl)carbenes, followed by the reversible switching of their physicochemical properties through simple protonation ( B base). Full size image Here we report that deprotonation of purposely designed aldiminium salt precursors allows for the efficient in situ generation of acyclic amino(aryl)carbenes. The latter intermediate species are then found to selectively and quantitatively dimerize into the corresponding diaminoalkenes. Such selectivity is rationalized by comparing the energy profiles of the dimerization process, relatively to putative competitive intramolecular C–H insertion pathways. Further application of this dimerization to hitherto unknown bis-amino(aryl)carbenes yields air-stable, non-dynamic, electron-rich N-PPV’s following a “dimerizing polymerization” pathway. Of particular interest and in contrast to classical PPV’s, the properties of N-PPV’s can readily be manipulated upon protonation, opening the avenue to PPV’s with tunable absorption or showing switchable “on-off” absorption. Acyclic MACs, and in particular amino(aryl)carbenes, have been accessed by different synthetic routes, including substitution of the phosphonio group at the carbene center of amino-phosphoniocarbene using aryl-lithium as nucleophiles, reduction of phosphonio aldiminium salts, or dechlorination of C-chloro iminiums with Hg(TMS) 2 [14] , [16] , [45] . Because related methodologies involve either rather sophisticated precursors or toxic reagents, we turned our attention to the deprotonation of aldiminium salts in presence of a strong base [11] . For that purpose, we kept in mind that methyl group at the nitrogen atom should be avoided to suppress any carbene to azomethine ylide isomerization [46] . The substitution pattern of the aryl moiety, especially at the ortho positions, has also been shown to dramatically influence the kinetic stability of the carbene, which eventually controls its deactivation pathways (dimerization versus C–H insertions) [11] , [46] , [47] . In-situ generation of amino(aryl)carbene 2a–c On this basis, mono-iminiums 1 , i.e. featuring a di-isopropylamino/phenyl ( 1a ), piperidyl/phenyl ( 1b ) or piperidyl/fluorenyl ( 1c ) substitution pattern, were selected and synthesized according to established procedures (Fig. 2a ) [48] , [49] . LiHMDS was initially investigated for the deprotonation of 1a-c at −80 °C in THF. Monitoring these reactions by 1 H NMR spectroscopy evidenced that quantitative conversions of 1a-c into the corresponding diaminoalkenes, 3a-c , were achieved, highlighting the high selectivity of those transformations. Upon purification, 3a-c were obtained in good yields (60–70%, see Supporting information for details) as a mixture of E/Z isomers in a molar ratio of 80/20 for 3a and 85/15 for 3b and 3c , respectively. Alternatively, a neutral organic strong base, such as phosphazene P 4 - t Bu, could also be successfully employed instead of LiHMDS, thus providing a transition metal-free synthetic route to 3a-c . Fig. 2: Reactivity of in situ generated mono- and bis-amino(aryl)carbenes. a Dimerization of mono-carbenes 2a-c and trapping of 2a. b Ortep drawing of the molecular structure of dimer 3 a - E . Hydrogen atoms are omitted for clarity. Carbon atoms are represented in gray and nitrogen atoms in blue. Thermal ellipsoids are shown at 50% probability. c In situ generation of bis-carbenes 8a-c and formation of the corresponding N-PPV’s 9a-c: iPr = isopropyl, Pip = piperidine, Ph = phenyl, Fluo = 9,9-dihexyl-9H-fluorene (see Fig. 1 ). d Size exclusion chromatography trace in THF of N-PPV 9b (M n = 3900 g mol −1 ; Đ = 2.05; calibration with PS standards). Full size image Characterization of 3a by X-ray diffraction analysis These compounds were thoroughly characterized by 1 H and 13 C NMR spectroscopy, but also by X-Ray diffraction analysis (see Supporting Information for details). In the case of 3a , single crystals could be grown from a pentane solution of 3a at −20 °C. Under those conditions, only the E-isomer was found to crystallize ( 3a–E ; Fig. 2b ). The asymmetric unit of 3a-E contains two independent molecules. However, only one molecule is described as they both have similar geometrical parameters (C 3 -N 1 and C 4 -N 2 bonds of 1.42 Å and 1.41 Å respectively; C=C bond of 1.359 Å and dihedral angles C 1 -C 2 -C 3 -C 4 of 68° and C 3 -C 4 -C 5 -C 6 of 62°). X-Ray analysis revealed that the C 3 =C 4 bond distance (1.354 Å) was slightly longer than that of trans-stilbene (1.318 Å), while the C 3 -N 1 /C 4 -N 2 bond lengths (1.41 Å and 1.41 Å, respectively) proved shorter than a single C-N bond (1.469 Å). These data thus suggested some interaction between the lone pairs on nitrogen atoms and the central double bond in the solid state [50] , [51] . Furthermore, in comparison with the near planarity of trans-stilbene (dihedral angle C 1 -C 2 -C 3 -C 4 of 5°), phenyl groups were found significantly tilted in 3a-E (dihedral angles C 1 -C 2 -C 3 -C 4 of 68° and C 3 -C 4 -C 5 -C 6 of 69°), to accommodate the steric congestion imposed by the bulky di-isopropylamino groups. Characterization of 3 by UV/Vis spectroscopy analysis In chloroform solution, this interaction between the amino groups and the central C=C double remained, as evidenced by the strong absorption in the 388–440 nm range observed by UV/Vis analysis of 3a-c (see Supporting Information for details), which is red-shifted in comparison with that of trans-stilbene ( λ max = 322 nm) [51] . According to DFT calculations (B3LYP/def2-SVP), this absorption corresponds to the HOMO-LUMO transition, the HOMO being mainly localized both on π C=C and n N − orbitals and the LUMO being a combination of π* C=C with π* C=C(phenyl) orbitals (see Supplementary Figs. 22 , 23 and Supplementary Table 2 for details). 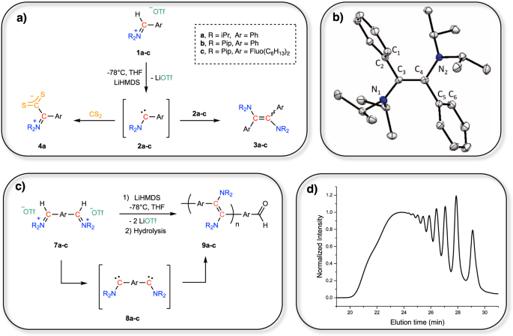Fig. 2: Reactivity of in situ generated mono- and bis-amino(aryl)carbenes. aDimerization of mono-carbenes 2a-c and trapping of 2a.bOrtep drawing of the molecular structure of dimer 3a-E. Hydrogen atoms are omitted for clarity. Carbon atoms are represented in gray and nitrogen atoms in blue. Thermal ellipsoids are shown at 50% probability.cIn situ generation of bis-carbenes 8a-c and formation of the corresponding N-PPV’s 9a-c: iPr = isopropyl, Pip = piperidine, Ph = phenyl, Fluo = 9,9-dihexyl-9H-fluorene (see Fig.1).dSize exclusion chromatography trace in THF of N-PPV 9b (Mn= 3900 g mol−1;Đ= 2.05; calibration with PS standards). Trapping of carbene 2a with CS 2 Despite several attempts to characterize 2a by monitoring the deprotonation of 1a by 13 C NMR spectroscopy at −80 °C, no carbene could be identified, as the characteristic low-field signal expected around 300 ppm in the 13 C NMR spectrum could not be detected. Nevertheless, betaine 4a , resulting from the trapping of carbene 2a with CS 2 (Fig. 2a ), was fully characterized by 1 H, 13 C NMR, and X-Ray diffraction analyses (see Supplementary Information), which strongly supports the in situ generation of 2a . DFT calculation Although the dimerization of (cyclic) diaminocarbenes has been theoretically investigated [13] , [15] , [17] , data concerning MACs, and particularly amino(aryl)carbenes, are lacking. Therefore, to gain some insight into the selective dimerization of carbenes 2a , relative to putative intramolecular C-H insertion reactions [47] , DFT calculations were carried out on the direct dimerization of 2a , as well as on the intramolecular C-H insertion of 2a into CHiPr and CH 3 iPr at the B3LYP/def2-SVP level of theory. The β-H elimination of propene from i Pr 2 N-substituted carbene 2a was also investigated in the Supplementary Information . 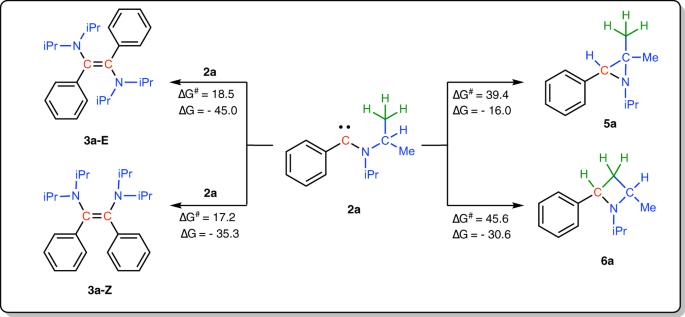Fig. 3: Theoretical investigation of the reactivity of 2a. General view of the energetic profiles for the dimerization of carbene 2a into diaminoalkenes 3a-E/Z and for the putative intramolecular CHiPr and CH3iPr insertion reactions (see Supporting Information for details), at the B3LYP/def2-SVP level of theory; Gibbs free energy are expressed in kcal. mol−1. Furthermore, computational details, as well as in depth discussion of structural parameters relative to transition states involved in those processes can be found in the Supplementary Information . As anticipated, carbene 2a was found to possess a singlet ground state that lays 18.5 kcal mol −1 below the triplet state. The C carbene -N bond proved short (1.304 Å) and the nitrogen atom was found in a planar environment (Σ N = 360.0°), indicating a strong interaction between the nitrogen lone pair and the carbene empty orbital. 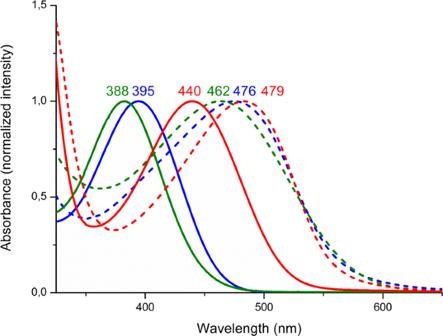Fig. 4: UV/Vis spectrometry of dimers 3 and corresponding N-PPV’s 9 in CHCl3. Solid lines, green3a, blue3b, red3c; dashed lines, green9a, blue9b, red9c. Furthermore, the acute NCC Ph angle (124.2°) and the long C-C Ph bond distance of 1.457 Å attested that the phenyl group merely behaved as a mesomeric spectator. Investigation of the dimerization of 2a Dimerization reactions of 2a into the corresponding diaminoalkenes 3a-E and 3a-Z were next computed, as summarized in Fig. 3 (see also the Supplementary Fig. 24 and Supplementary Table 5 ). 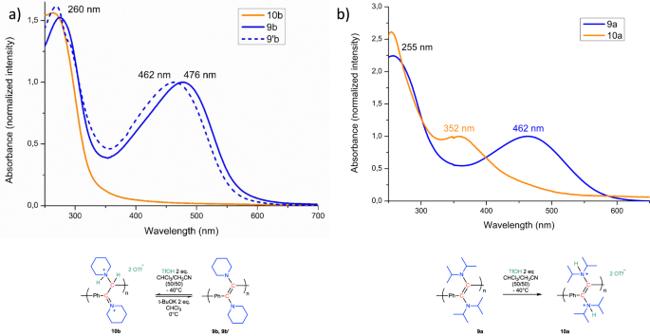Fig. 5: Switching of the absorption of N-PPV’s 9. aProtonation of N-PPV9b(solid blue line) using TfOH and subsequent deprotonation of polymer10b(solid orange line) in presence of t-BuOK leading to N-PPV9’b(dashed blue line), along with their respective UV spectra (9b,9’band10b).bProtonation of N-PPV9ausing TfOH and formation of poly(cation)10aand their corresponding UV spectra (9aand10a). From a kinetic point of view, moderate activation barriers (18.5 and 17.2 kcal mol −1 for 2a → 3a-E and 2a → 3a-Z , respectively) were calculated. In addition, both transformations were predicted strongly exergonic (Δ G = −45.0 and −35.3 kcal mol −1 for 2a → 3a-E and 2a → 3a-Z , respectively), the relative stability of 3a-E vs. 3a-Z being in agreement with experimental observations ( 3a-E and 3a-Z being the thermodynamic and kinetic product, respectively). Fig. 3: Theoretical investigation of the reactivity of 2a. General view of the energetic profiles for the dimerization of carbene 2a into diaminoalkenes 3a-E/Z and for the putative intramolecular CHiPr and CH 3 iPr insertion reactions (see Supporting Information for details), at the B3LYP/def2-SVP level of theory; Gibbs free energy are expressed in kcal. mol −1 . Full size image Investigation of putative insertion reactions of 2a In the case of the putative transformations of 2a into cyclopropane 5a and cyclobutane 6a , via carbene insertion into CHiPr and CH 3 iPr, respectively, both reactions were predicted to be highly exergonic (−16.0 and −30.6 kcal mol −1 , respectively). However, activation barriers of 39.4 kcal mol −1 and 45.6 kcal mol −1 were calculated for the insertion of 2a into CHiPr and into CH 3 iPr, respectively (see Fig. 3 and the Supplementary Fig. 25 and Supplementary Table 6 ). In other words, both insertion reactions proved prohibitively too high to compete with the dimerization process under our experimental conditions. Dimerizing polymerization of in-situ generated bis-carbenes 8a-c The high conversion and complete selectivity in favor of the formal dimerization of 2a-c into the corresponding diaminoalkenes 3a-c prompted us to design original bis-aldiminium salts 7a-c and to investigate their deprotonation (see Fig. 2c ). Indeed, the resulting in situ generated bis-carbenes 8a-c would thus serve as difunctional monomeric substrates and would lead to an original class of PPV’s, namely amino-PPV’s (N-PPV’s), which can be hardly accessed by other means, here following a dimerizing step-growth polymerization pathway. Bis-aldiminiums 7a-c were thus prepared by adapting the procedures followed for the preparation of mono-iminiums 1a-c . Characterization of N-PPV’s 9a-c Bis-aldiminiums 7a-c displayed similar NMR spectra, with very few signals due to their symmetrical nature. For instance, while 7a possesses 34 protons, only 6 different signals were observed in its 1 H NMR spectrum. Most notably, the characteristic CH iminium appeared as the most downfield signal at 9.5 ppm (172 ppm in 13 C NMR) and only a singlet at 7.86 ppm, integrating for 4H, was observed for the para -disubstituted phenyl group. Upon deprotonation of 7a-c using either LiHMDS or P 4 - t Bu in THF, a gradual red color appeared, suggesting the formation of the targeted conjugated N-PPV’s 9a-c (Fig. 2c ). Remarkably, those polymers proved air-stable and do not exhibit any dynamic behavior, in contrast to conjugated polymers derived from bis-benzimidazolylidenes [29] , [30] , [31] . This difference also highlights how the substitution pattern of the carbene center dictates, not only the structure but also the properties of the resulting polymers. SEC analysis revealed typical traces of a step-growth polymerization process (see Fig. 2d for a representative SEC trace), with multimodal distributions composed of discrete peaks corresponding to oligomers: M n = 3000 (dispersity, Đ = 2.08), 3900 ( Đ = 2.05), and 5200 g mol −1 ( Đ = 2.60) for 9a , 9b, and 9c , respectively (Supplementary Figs. 4 – 6 ). Importantly, molar masses of 9a and 9c determined by MALDI ToF mass spectrometry were found in rather good agreement with values delivered by SEC, with DP = 5-6 and DP = 10 for 9a and 9c , respectively (see Supplementary Figs. 20 and 21 ). Furthermore, 3 distinct populations could be identified, in the case of 9c , with different chain ends. Among these, one population corresponded to the expected bis-aldehyde-terminated N-PFV, owing to the hydrolysis of both iminium/carbene chain-ends chain during workup, while another population was ascribed to a N-PFV carrying an iminium and an aldehyde chain end. Interestingly, cyclic N-PFV structures consisting of 3–9 repeating units were also identified in the MALDI ToF mass spectrum of 9c (see Supplementary Fig. 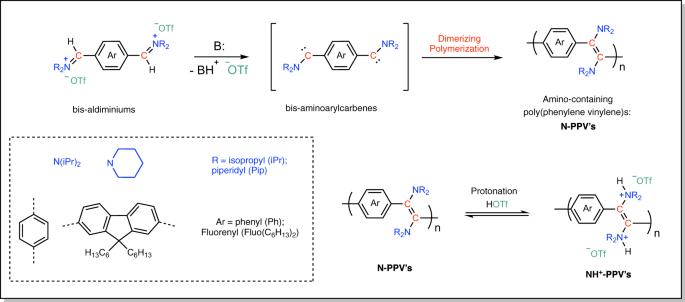20 ). In comparison with the 1 H NMR spectra of diaminoalkenes 3a-c , N-PPV’s 9a-c displayed signals with similar chemical shifts, but showed evident broadening due to their polymeric nature. The only sharp signal observed at 10.0 ppm in the 1 H NMR spectrum of 9a-c corresponded to aldehyde end-groups, arising from the hydrolysis of carbene/iminium chain ends during workup in air, in agreement with structures determined by mass spectrometry. Importantly, similar E/Z ratios of 80-85/20-15 were determined for both 9 and 3 , suggesting independent reactivity of each carbene site in the bis-carbene monomers. Fig. 1: Synthetic strategy to amino-poly(phenylene vinylene)s (N-PPV’s). NPPV’s via dimerizing polymerization of in situ generated bis-amino(aryl)carbenes, followed by the reversible switching of their physicochemical properties through simple protonation (Bbase). It should be noted that higher molecular weight N-PPV’s could not be reached despite the investigation of several experimental conditions, including variations in the nature of both the solvent and the base, and in the concentration (see Supplementary Table 1 ). Those limitations may stem from the building of steric hindrance around the carbene center upon repeated dimerization reactions. In parallel, DFT calculation suggested that β-H elimination of propene from iPr 2 N-substituted carbene 2a could compete with the dimerization reaction (Δ G = −18.5 kcal mol −1 and Δ G # = 19.1 kcal mol −1 ; Supplementary Figure 26 and Supplementary Table 7 ). In the case of piperidine-substituted carbenes, such a deactivation pathway should not be operative owing to the geometrical constraint imposed by the cyclic structure of the stabilizing amino group. Finally, the increased conjugation in polymers 9a-c , respectively to diaminoalkenes 3a-c , could also be appreciated from the red-shift (43–76 nm) of the maximum absorption by UV/Vis analysis (Fig. 4 ). By analogy with molecular diaminoalkenes 3a-c , the interaction between the amino groups and the C=C bond in N-PPV’s 9a-c resulted in a bathochromic effect on the λ max compared to the parent PPV (440–483 nm vs. 400–420 nm for N-PPV’s and PPV’s respectively) [52] , [53] . Furthermore, the large stoke shifts observed (see Supplementary Figs. 17 – 19 ) are promising considering their possible integration into light-emitting devices. Fig. 4: UV/Vis spectrometry of dimers 3 and corresponding N-PPV’s 9 in CHCl 3 . Solid lines, green 3a , blue 3b , red 3c ; dashed lines, green 9a , blue 9b , red 9c . Full size image Film-forming properties of N-PPV’s The film-forming properties of N-PPV’s 9 were also briefly investigated. Gratifyingly, while the formation of PPV’s film generally requires high molar mass, a homogeneous film with a thickness of 85 nm could be prepared by spin-coating a 15 mg/mL chloroform solution of 9c onto a glass substrate (Supplementary Figs. 1 – 4 ). The film stability was evidenced by AFM and optical microscopy. Tuning the absorption of N-PPV’s 9 by protonation While tuning the properties of classical PPV’s is challenging, the presence of amino groups in α-position of the C=C bonds in N-PPV’s 9a-c provides facile means to vary the properties of this organic polymeric platform, upon chemical post-modification (Fig. 5 ). Fig. 5: Switching of the absorption of N-PPV’s 9. a Protonation of N-PPV 9b (solid blue line) using TfOH and subsequent deprotonation of polymer 10b (solid orange line) in presence of t-BuOK leading to N-PPV 9’b (dashed blue line), along with their respective UV spectra ( 9b , 9’b and 10b ). b Protonation of N-PPV 9a using TfOH and formation of poly(cation) 10a and their corresponding UV spectra ( 9a and 10a ). Full size image Thus, in a preliminary experiment, treatment of 9b with 2 eq. of TfOH at −40 °C in a CH 3 CN/CHCl 3 mixture (50/50) led to the disappearance of the maximum absorption at 476 nm, suggesting that the conjugation was disturbed in 10b (see Fig. 5a ). Interestingly, this process was found to be fully reversible and the maximum absorption could be recovered in 9’b upon deprotonation of 10b using t- BuOK at 0 °C. The identity of 9’b was also confirmed by 1 H NMR analysis. While a similar behavior was observed with 9c , a completely different scenario was evidenced with 9a . In the latter case, the maximum absorption initially at 462 nm was blue-shifted to 352 nm upon protonation (Fig. 5b ). This different behavior may be surprising as 9a and 9b only differ by the nature of the amino substituents on the C=C bond (di-isopropylamino vs . piperidine in 9a and 9b , respectively). To gain some insight into the different behavior of 9a and 9b , protonation of the corresponding molecular dimers, 3a and 3b , was then carried out using 2 eq. of TfOH (see Supplementary Information ). According to X-ray diffraction analysis, protonation of 3a occurred at both nitrogen atoms, the C=C bond being preserved. In sharp contrast, 3b underwent protonation at only one nitrogen atom and at the enamine carbon atom, ultimately leading to a dicationic compound without C=C bond (see Supplementary Information for details). By analogy, we thus hypothesized that protonation of N-PPV’s 9a and 9b would lead to conjugated poly(ammonium) derivative 10a (Fig. 5b ) and non-conjugated 10b (Fig. 5a ), respectively, in agreement with a blue-shift and the disappearance of the λ max in the UV/vis spectrum of 9a and 9b upon protonation. Overall, this study demonstrates that weakly kinetically stabilized acyclic amino(aryl)carbenes undergo a facile and highly selective dimerization reaction, yielding the corresponding diaminoalkenes. Of particular interest, in situ generated bis-amino(aryl)carbenes lead to the formation of air-stable N-PPV’s by a dimerizing step-growth polymerization route. Importantly, N-PPV’s reported herein cannot be prepared by traditional routes. Furthermore, and in contrast to more conventional PPV’s, the presence of amino groups adjacent to the C=C double bonds in N-PPV’s allows their properties to be manipulated in different ways upon protonation, depending on the nature of the substituent on the nitrogen atoms. Thus, this work could pave the way toward PPV’s featuring tunable absorption and/or to sensor-type materials thanks to the ability of N-PPV’s to readily form stable films. Future work is also underway to expand the synthetic interest of this under-explored class of mono-amino carbenes in the context of polymer chemistry, through a careful and more systematic design of the substitution pattern of the carbene center. Materials THF and Et 2 O were dried over sodium/benzophenone and distilled prior to use. Dichloromethane, chloroform and pentane were dried over CaH 2 and distilled prior to use. Acetonitrile solvent was dried using a MBraun Solvent Purification System (model MB-SPS 800) equipped with alumina drying columns. Benzaldehyde (Alfa Aesar, 98%) was dried over CaH 2 , distilled and stored under argon. n -Butyllithium solution 11 M in hexanes, Lithium bis(trimethylsilyl)amide, Phosphazene (P 4 - t Bu) 0.8 M in hexane and terephthalaldehyde were purchased from Sigma-Aldrich and used without further purification. Diisopropylformamide (Alfa Aesar) and piperidinoformamide (Sigma Aldrich) were stored under argon over activated molecular sieves 4 Å. Trifluoromethanesulfonic acid (TCI), Trifluoromethanesulfonic anhydride (ABCR), and benzaldehyde (Alfa Aesar) were distilled prior to use. Phenyllithium 1.9 M in di-n-butyl ether was purchased from Alfa Aesar and used without purification. Instrumentation NMR spectra were recorded on a Bruker Avance 400 (1H, 13 C, 19 F, 400.2, 100.6, and 376.53 MHz, respectively) in appropriate deuterated solvents. Molar masses were determined by size exclusion chromatography (SEC) in THF + 10% of Et 3 N [54] , [55] , [56] (1 mL/min) with trichlorobenzene as flow marker, using both refractometric (RI) and UV detectors. Analyses were performed using a three-column TSK gel TOSOH (G4000, G3000, G2000) calibrated with polystyrene standards. HRMS were recorded on various spectrometer: a Waters Q-TOF 2 spectrometer and a GCT premier water mass spectrometer in the chemical ionization mode. Melting point were determined by using a Stuart Scientific SMP3 apparatus. Ultraviolet–visible spectra were collected on a thermostated UV/Vis Spectrometer (Agilent Carry 4000). Fluorescence spectra were obtained via Spectrofluorimeter (Jasco FP-8500ST). XRay structures were done on a Rotating Anode Rigaku FRX 3 kW with microfocus (Hybrid Dectris Pilatus 200 K pixel detector). Synthesis of aldiminium salt precursors A typical procedure to synthesize benzylidenediisopropyliminium triflate, 1a , is as follows. Following the Alder’s route : To a stirred solution of diisopropylformamide (1.38 mL, 9.5 mmol) in dry ether (50 mL) cooled at −78 °C was added phenyllithium (1.9 M, 7.9 mL) dropwise and the resulting mixture was stirred at this temperature for 30 min then at room temperature for 1 h. Then, to the reaction mixture cooled at −78 °C was added trifluoromethanesulfonic anhydride and the mixture was stirred for 1 h at this temperature then for 2 h at room temperature. The precipitated solid was filtered under argon and washed with dry ether (3 × 5 mL) and THF (3 × 5 mL) and dried under vacuum to obtain compound 1a , as white crystals (2.1 g, 70%). Following the Schroth’s route : To a stirred solution of benzaldehyde (1 mL, 10 mmol) and 1-(trimethylsilyl) diisopropylamine (1.45 g, 10 mmol) in dry ether (50 mL), TMSOTf (1.8 mL, 10 mmol) was added dropwise at room temperature and the resulting mixture was stirred at the same temperature for 6 h under inert atmosphere. The precipitated solid was filtered under inert atmosphere and dried under vacuum to obtain compound 1a as white crystals (2.32 g, 70%). See the Supplementary Information for a complete characterization. Dimerization reaction from monofunctional adiminium salts A typical procedure leading to the diamino-containing alkenes, 3a , is as follows. Using P 4 - t Bu base : To a stirred solution of 1a (0.1 g, 0.3 mmol) in THF (6 mL) cooled at −78 °C, P 4 - t Bu base (0.38 mL, 0.3 mmol, 0.8 M in hexanes) was added and the resulting mixture was stirred at this temperature for 1 h followed by 24 h at room temperature. The solvent was evaporated under reduced pressure and the reaction mixture was diluted with pentane (20 mL) and passed through a short column of basic alumina. The final compound 3a (0.034 g, 60%) was obtained as a yellow solid. Single crystals were grown from the slow evaporation of a pentane solution of 3a at −20 °C. Using LiHMDS base : 1a (0.1 g, 0.3 mmol) and LiHMDS (50 mg, 0.3 mmol) were dissolved in cold THF (6 mL, −78 °C). The resulting mixture was stirred at this temperature for 1 h followed by 24 h at room temperature. The solvent was evaporated under reduced pressure and the reaction mixture was diluted with pentane (20 mL) and passed through a short column of basic alumina. The final compound 3a (0.034 g, 60%) was obtained as a yellow solid. Single crystals were grown from the slow evaporation of a pentane solution of 3a at −20 °C. See the Supplementary Information for a complete characterization. Synthesis of amino-containing poly(phenylene vinylene)s (N-PPV’s) by dimerizing polymerization from in situ generated bis-aminoaryl carbenes A typical procedure for achieving N-PVV 9a is as follows. To a stirred solution of 7a (0.300 g, 0.5 mmol) in THF (2 mL) cooled at −78 °C P 4 -tBu base (1.38 mL, 1.1 mmol, 0.8 M in hexanes) was added and the resulting mixture was stirred at this temperature for 1 h followed by 24 h at room temperature. After the solvent was removed under reduced pressure, the mixture was washed with MeOH (10 mL) to remove the phosphazenium salts. The resulting mixture was dissolved in CHCl 3 (15 mL) and filtered to remove the insoluble compounds. After evaporation of the organic solvent, the mixture was purified by precipitation using CHCl 3 and MeOH at −10 °C to obtain the desired polymer 9a as a dark red solid (80 mg, 60%). See the Supplementary Information for a complete characterization and for an optimization study. Post-chemical modification of N-PPV’s A typical protonation of N-PPV 9 is as follows. To a solution of polymer precursor 9b (0.134 g, 0.50 mmol) in CH 3 CN/CHCl 3 (50/50) cooled at −40 °C, TfOH (184.2 μL, 2.2 mmol) was added dropwise. The resulting mixture was warm to room temperature overnight and the organic solvent was evaporated to give the compound 10b , namely, poly(7,8-bispiperidinium-1,4-phenylenevinylene) bis-triflate: (99%, 0.245 g); UV/Vis (CH 3 CN) λ max = 254 nm. Deprotonation of polymer 10b is as follows. To a stirred solution of 10b (0.054 g, 0.1 mmol) in CH 3 CN/CHCl 3 (50/50) cooled at 0 °C, t -BuOK (0.021 g, 0.2 mmol) was added. The reaction was warmed to room temperature overnight, and the solvents were removed under reduced pressure and the resulting mixture was extracted with CHCl 3 leading to the final polymer 9b (0.048 g, 89%).